Wnt5a uses CD146 as a receptor to regulate cell motility and convergent extension Dysregulation of Wnt signalling leads to developmental defects and diseases. Non-canonical Wnt signalling via planar cell polarity proteins regulates cell migration and convergent extension; however, the underlying mechanisms are poorly understood. Here we report that Wnt5a uses CD146 as a receptor to regulate cell migration and zebrafish embryonic convergent extension. CD146 binds to Wnt5a with the high affinity required for Wnt5a-induced activation of Dishevelled (Dvl) and c-jun amino-terminal kinase (JNK). The interaction between CD146 and Dvl2 is enhanced on Wnt5a treatment. Mutation of the Dvl2-binding region impairs its ability to activate JNK, promote cell migration and facilitate the formation of cell protrusions. Knockdown of Dvls impairs CD146-induced cell migration. Interestingly, CD146 inhibits canonical Wnt signalling by promoting β-catenin degradation. Our results suggest a model in which CD146 acts as a functional Wnt5a receptor in regulating cell migration and convergent extension, turning off the canonical Wnt signalling branch. Extensive cell movements occur during the embryonic development of vertebrates. Cell migration allows different types of cells to find their proper positions in which they can function appropriately. Convergent extension (CE) is the main driving force in shaping the dorsal body axis, driving involution and in leading to the asymmetric closure of the blastopore and the formation of an elongated body [1] . These processes are tightly regulated by conserved signalling pathways such as Wnt, bone morphogenic proteins and Hedgehog (Hh) signalling pathway [2] , [3] . Dysregulation of these signalling pathways may trigger developmental defects or diseases. The Wnt family is a large family of protein ligands that affect various processes such as embryonic patterning, cell polarity formation, cell motility and cell fate specification. Wnt signalling is also involved in the homoeostasis and self-renewal of stem cells as well as in tumorigenesis [4] . Wnt signalling pathways are classified according to the stability of cytoplasmic β-catenin [5] into canonical and non-canonical pathways. Canonical Wnt ligands, such as Wnt1 and Wnt8, bind to the receptor Frizzled (Fz) and co-receptors LRP5/6 to recruit Dishevelled (Dvls) and Axin and subsequently disrupt the β-catenin degradation complex. The stabilized β-catenin then translocates into the nucleus to regulate the expression of the target genes of the co-activator of T cell factor (TCF/Lef) (ref. 6 ). Wnt5a-activated signalling is ascribed to non-canonical Wnt signalling, which is further divided into several branches such as Wnt/planar cell polarity (PCP), Wnt/Ror2 and Wnt/Ca2+ signalling. Wnt/PCP signalling is the best defined of these branches. Polarity or PCP is a fundamental property of many cells and has critical roles in regulating CE during vertebrate gastrulation, orientation of bird feathers and mammal hair as well as in the polarization of inner ear hair cells that is essential for hearing and balance [7] . Molecular and genetic studies have indicated that the Wnt receptor Fz is important in the PCP pathway. Fz relays Wnt signalling to a cytoplasmic scaffold protein Dvl, and then activates small GTPase and c-jun amino-terminal kinase (JNK), finally modulating cytoskeleton rearrangement [8] . In addition to Fz, several other receptors, including Ror2, Flamingo and Ryk, are involved in the non-canonical Wnt pathway [7] , [9] . In some cases, depending on the receptor context, non-canonical Wnt ligands or receptors such as Wnt5a or Ror2 can inhibit canonical Wnt signalling [10] , [11] . CD146 is an adhesion molecule that belongs to a subgroup of the immunoglobulin (Ig) superfamily and consists of a characteristic V-V-C2-C2-C2 Ig-like extracellular domain (ECD) structure, a transmembrane domain and a short cytoplasmic region [12] . CD146 was first identified as a marker for melanoma progression [13] . Later on, CD146 was also identified as a factor in angiogenesis, and tumour cell invasion and migration [14] , [15] , [16] , [17] . We have previously reported that CD146 regulates cell migration through cytoskeleton proteins by activating the small GTPase RhoA [18] . However, the underlying mechanism of CD146 has remained elusive. In this study, we show that CD146 interacts with Wnt5a and acts as a Wnt5a receptor in regulating the migration and polarity of mammalian cells, and the CE of gastrulation in zebrafish. To fulfill these functions, CD146 activates non-canonical Wnt signalling via a Wnt/Dvl/JNK cascade and inhibits canonical Wnt signalling by promoting β-catenin degradation. CD146 binds to Wnt5a To identify potential binding partners of CD146, we employed a yeast two-hybrid assay. Our screen identified Wnt5a as a binding protein of CD146. To examine the functional interaction between Wnt5a and CD146, we next performed a cell surface-binding assay using HEK293T cells [19] . Cells were transfected with Flag-tagged CD146, Fz5 or Fz7 (two well-known Wnt receptors as positive controls) and an empty vector as a negative control [20] . Results showed that after incubation with Myc-Wnt5a conditional medium (CM), Wnt5a bound to cells transfected with CD146, Fz5 or Fz7, whereas no Wnt5a binding was detected for empty vector-transfected cells ( Fig. 1a ). To evaluate whether the binding between Wnt5a and CD146 is direct, we performed pull-down assays by incubating recombinant Wnt5a protein with the purified Fc-fused CD146 ECD (Fc-CD146/ECD), Fc-fused Fz5 ECD (Fc-Fz5/ECD, positive control) and Fc (negative control). After sedimentation with protein A beads, Wnt5a was detected in both Fc-CD146/ECD and Fc-Fz5/ECD precipitates but not in the Fc control ( Fig. 1b ), indicating that CD146 binds Wnt5a directly. 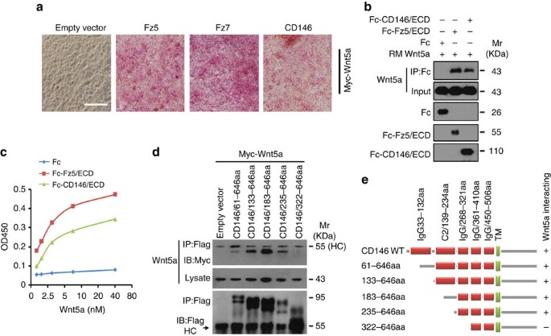Figure 1: CD146 binds Wnt5a with high affinity. (a) Wnt binds CD146 at the cell surface.Flag-CD146was transfected into HEK293T cells for 36 h and incubated with Myc-Wnt5a CM for an additional 3 h. Staining was performed as described in the Methods (scale bar, 150μm).xFz7andhFz5were used as positive controls, whereas an empty vector was used as a negative control. (b) The CD146 ECD (CD146/ECD) binds Wnt directly. Fc-fused CD146/ECD, Fz5/ECD, or human Fc alone incubated with protein A beads were incubated with recombinant Wnt5a (100 ng) for 1 h at 4 °C. Bound proteins were washed and subjected to western blotting. (c) CD146 binds Wnt5a with high affinity. Different concentrations of Wnt5a were added to wells coated with 0.4 mg ml−1of Fc-CD146/ECD, Fc-Fz5/ECD or Fc and enzyme-linked immunosorbent assay was performed as described in Methods. (d) The third Ig-like region is critical for CD146 binding to Wnt5a. 1 μg N-terminal Flag-tagged CD146 (as indicated inFig. 1e) was co-expressed with 1 μg Myc-tagged Wnt5a in HEK293T cell for 36 h, cells lysate was subjected to co-IP assay with M2 anti-Flag antibody and western blot performed as described in Methods section. (e) Schematic diagram of different Ig-like regions of truncated CD146 and their interactions with Wnt5a. Figure 1: CD146 binds Wnt5a with high affinity. ( a ) Wnt binds CD146 at the cell surface. Flag-CD146 was transfected into HEK293T cells for 36 h and incubated with Myc-Wnt5a CM for an additional 3 h. Staining was performed as described in the Methods (scale bar, 150μm). xFz7 and hFz5 were used as positive controls, whereas an empty vector was used as a negative control. ( b ) The CD146 ECD (CD146/ECD) binds Wnt directly. Fc-fused CD146/ECD, Fz5/ECD, or human Fc alone incubated with protein A beads were incubated with recombinant Wnt5a (100 ng) for 1 h at 4 °C. Bound proteins were washed and subjected to western blotting. ( c ) CD146 binds Wnt5a with high affinity. Different concentrations of Wnt5a were added to wells coated with 0.4 mg ml −1 of Fc-CD146/ECD, Fc-Fz5/ECD or Fc and enzyme-linked immunosorbent assay was performed as described in Methods. ( d ) The third Ig-like region is critical for CD146 binding to Wnt5a. 1 μg N-terminal Flag-tagged CD146 (as indicated in Fig. 1e ) was co-expressed with 1 μg Myc-tagged Wnt5a in HEK293T cell for 36 h, cells lysate was subjected to co-IP assay with M2 anti-Flag antibody and western blot performed as described in Methods section. ( e ) Schematic diagram of different Ig-like regions of truncated CD146 and their interactions with Wnt5a. Full size image To measure binding affinity between Wnt5a and CD146, we then added different concentrations of Myc-Wnt5a from the CM to 96-well plates coated with Fc-CD146-ECD, Fc-Fz5-ECD or Fc. Enzyme-linked immunosorbent assay results showed that absorption values at 450 nm increased with increasing Wnt5a concentration. The binding affinity was high, that is, 10 −9 M ( Fig. 1c ). The binding activity between Wnt5a and CD146 was comparable to that between Wnt5a and its known receptor Fz5, while no binding was observed with Fc alone. To further validate the interaction between Wnt5a and CD146, Myc-Wnt5a and Flag-CD146 were co-expressed transiently in HEK293T cells. The interaction between CD146 and Wnt5a was verified by co-immunoprecipitation (co-IP; Supplementary Fig. S1a ). To determine the region of CD146 involved in binding to Wnt5a, we generated a series of N-terminal Flag-tagged CD146 mutants with different Ig-like region truncations ( Fig. 1e ). Co-IP assay showed that there is no interaction between Wnt5a and (322-646aa/CD146) mutant, indicating that the third Ig-like region of CD146 is critical for its binding to Wnt5a ( Fig. 1d ). Further, the co-localization of CD146 and Wnt5a at the cell surface was demonstrated by immunostaining. However, no overlapping expression between Wnt5a and the (322-646aa/CD146) mutant was detected, which is consistent with co-IP results ( Supplementary Fig. S1b ). To clarify whether CD146 also binds to other Wnt ligands, Myc-Wnt1 or Myc-Wnt3a plasmids were co-expressed with CD146 in HEK293T cells. Co-IP results showed that CD146 binds to Wnt1 or Wnt3a, which is similar to non-canonical Wnt receptor Ror2 ( Supplementary Fig. S2a ). Our immunostaining results suggest that CD146 co-localizes with Wnt1 or Wnt3a at the cell surface ( Supplementary Fig. S2b ). CD146 binds to Wnt3a with high affinity, which is comparable to that of Fz5 ( Supplementary Fig. S3 ).Taken together, these results suggest that CD146 is a potential receptor of Wnt. CD146 is essential for Wnt5a-induced cell migration Wnt5a/Dvl/JNK signalling is the best-studied non-canonical Wnt branch in regulating cell motility. To analyse the role of CD146 in Wnt5a-induced cell motility, CD146-specific short interfering RNAs (siRNAs) was employed to knock down endogenous CD146 in human umbilical vein endothelial cells (HUVECs) ( Fig. 2a ). With depletion of CD146, the motility of HUVECs decreased was very limited compared with that of HUVECs transfected with control siRNA. Wnt5a induced migration of significantly higher numbers of cells compared with the non-treated group, whereas knockdown of endogenous CD146 largely impaired Wnt5a-induced cell migration. To validate that the loss of CD146 impairs Wnt5a-induced cell migration, we introduced an siRNA-resistant form of CD146 back into CD146-depleted HUVECs. Cell migration results indicated that addition of CD146 rescued Wnt5a-induced cell motility ( Fig. 2a ), confirming that CD146 is crucial for Wnt5a-induced cell motility. 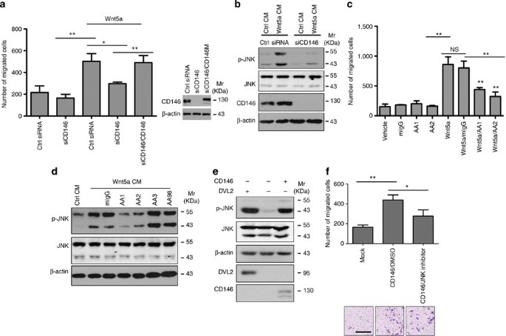Figure 2: CD146 is essential for Wnt5a-induced endothelial cell migration and JNK activity. (a) Knockdown of CD146 blocks Wnt5a-induced HUVEC migration; 5000 HUVECs depleted of CD146 were seeded in 8 mm transwell plates and incubated with Wnt5a or control. Knockdown efficiency and the expression level of siRNA-resistant form of CD146 were determined by western blotting, and migrated cells were stained and counted. Data are presented as mean values±s.d. of three experiments. Significant difference was determined by Student’st-test (*P<0.05; **P<0.01). (b) Knockdown of CD146 inhibits Wnt5a-induced JNK activity. HUVECs were transfected with CD146 siRNA or control siRNA for 48 h. Transfected cells were treated with Wnt5a or control CM for a further 1 h, and the phosphorylation of JNK was assessed by western blotting. β-actin was used as a loading control. (c) CD146-specific antibodies AA1 and AA2 block Wnt5a-induced HUVECs migration. 6,000 cells were pre-incubated with 50 μg ml−1mIgG, AA1 or AA2 for 1 h followed by addition of Wnt5a CM. Cells were cultured for 10 h, and migrated cells were stained and counted. Data are presented as mean values±s.d. of three experiments. Significant difference was determined by Student’st-test (**P<0.01; NS, no significant difference). (d) CD146-specific antibodies AA1 and AA2 block Wnt5a-induced JNK activity. HUVECs were pretreated with antibodies against the ECD of CD146 for 4 h, Wnt5a-induced JNK activity was determined by western blotting using P-JNK antibodies. β-actin was used as a loading control. (e) CD146 activates JNK. HEK293T cells were collected with ectopic expressed CD146 at 36 h and cell lysate was subjected to western blotting. JNK activity was demonstrated with antibody against p-JNK. Dvl2 and empty vector-transfected cells were used as positive and negative controls, respectively. β-actin was used as a loading control. (f) JNK inhibitor blocks CD146-promoted cell migration. CD146-HEK293T cells or mock cells seeded in 8 mm transwell plates were incubated with 10 mm JNK inhibitor SP600125or dimethyl sulphoxide. Migrated cells were stained and counted (scale bar, 150 μm). Data are presented as mean values±s.d. of three experiments. Significant difference was determined by Student’st-test (*P<0.05; **P<0.01). Figure 2: CD146 is essential for Wnt5a-induced endothelial cell migration and JNK activity. ( a ) Knockdown of CD146 blocks Wnt5a-induced HUVEC migration; 5000 HUVECs depleted of CD146 were seeded in 8 mm transwell plates and incubated with Wnt5a or control. Knockdown efficiency and the expression level of siRNA-resistant form of CD146 were determined by western blotting, and migrated cells were stained and counted. Data are presented as mean values±s.d. of three experiments. Significant difference was determined by Student’s t -test (* P <0.05; ** P <0.01). ( b ) Knockdown of CD146 inhibits Wnt5a-induced JNK activity. HUVECs were transfected with CD146 siRNA or control siRNA for 48 h. Transfected cells were treated with Wnt5a or control CM for a further 1 h, and the phosphorylation of JNK was assessed by western blotting. β-actin was used as a loading control. ( c ) CD146-specific antibodies AA1 and AA2 block Wnt5a-induced HUVECs migration. 6,000 cells were pre-incubated with 50 μg ml −1 mIgG, AA1 or AA2 for 1 h followed by addition of Wnt5a CM. Cells were cultured for 10 h, and migrated cells were stained and counted. Data are presented as mean values±s.d. of three experiments. Significant difference was determined by Student’s t -test (** P <0.01; NS, no significant difference). ( d ) CD146-specific antibodies AA1 and AA2 block Wnt5a-induced JNK activity. HUVECs were pretreated with antibodies against the ECD of CD146 for 4 h, Wnt5a-induced JNK activity was determined by western blotting using P-JNK antibodies. β-actin was used as a loading control. ( e ) CD146 activates JNK. HEK293T cells were collected with ectopic expressed CD146 at 36 h and cell lysate was subjected to western blotting. JNK activity was demonstrated with antibody against p-JNK. Dvl2 and empty vector-transfected cells were used as positive and negative controls, respectively. β-actin was used as a loading control. ( f ) JNK inhibitor blocks CD146-promoted cell migration. CD146-HEK293T cells or mock cells seeded in 8 mm transwell plates were incubated with 10 mm JNK inhibitor SP600125or dimethyl sulphoxide. Migrated cells were stained and counted (scale bar, 150 μm). Data are presented as mean values±s.d. of three experiments. Significant difference was determined by Student’s t -test (* P <0.05; ** P <0.01). Full size image CD146 is essential for Wnt5a-induced JNK activity To further investigate the function of CD146 in relaying Wnt5a-induced signalling, we examined the phosphorylation of JNK, the downstream effector of Wnt5a-induced non-canonical Wnt signalling. Wnt5a activated JNK strongly and in a time-dependent manner, with activity reaching a peak at 1 h after treatment, whereas Wnt1 hardly had any effect ( Supplementary Fig. S4a ). However, on depletion of endogenous CD146, Wnt5a-activated JNK was suppressed ( Fig. 2b ). Moreover, the blocking antibodies (AA1 and AA2), which recognize the ECD of CD146 effectively inhibited Wnt5a-induced cell migration and JNK activation ( Fig. 2c,d ), probably through interfering with the interaction between CD146 and Wnt5a ( Supplementary Fig. S5 ). However, AA1/AA2 does affect cell adhesion ( Supplementary Fig. S6a ). Altogether, these results suggest that CD146 is essential for non-canonical Wnt5a-activated Wnt signalling. CD146 promotes cell migration by activating JNK CD146 has been identified as an inducer of cell migration. As CD146 binds Wnt5a with high affinity and is essential for Wnt5a-induced JNK activation and cell migration, we then evaluated whether CD146 can promote cell migration by activating JNK. When CD146 was expressed in HEK293T cells, JNK activity increased to a level comparable to that in Dvl2-transfected cells ( Fig. 2e ). To further investigate whether CD146 can activate non-canonical Wnt signalling JNK alone, the expression levels of Wnt5a and several Wnt receptors were examined by reverse transcriptase–PCR in HEK293T and HUVECs. Our results show that Wnt5a and Wnt receptors were expressed in those cells as reported [21] , [22] , [23] . Subsequently, specific siRNAs were employed to knock down the different Wnt receptors in HEK293T cells ( Supplementary Fig. S7b , Supplementary Tables S1 and S2 ). CD146 activated JNK efficiently in the absence of all those receptors except Fz4, which is involved in regulating Wnt/PCP signalling ( Supplementary Fig. S7a ) [24] . Knockdown of CD146 does not affect Fz5, Fz7 and Ror2-activated JNK ( Supplementary Fig. S8 ). Further, modulating the expression of CD146 does not alter the expression and subcellular localization of other Wnt4 receptors, such as Fz5, Fz7 and Ror2 in HEK293T cells ( Supplementary Figs S9 and S10 ) Thus, our results showed that CD146 activation of non-canonical Wnt signalling may work through cooperation with Fz4, although the mechanistic details involved will require further investigation. Further, we generated a HEK293T cell line that constitutively expressed CD146 (CD146-HEK293T). Cell motility assays indicated that ectopic expression of CD146 significantly promotes cell migration in HEK293T cells compared with mock cells ( Fig. 2f ) Immunoblotting showed that JNK phosphorylation was upregulated in CD146-HEK293T cells compared with HEK293T cells transfected with an empty vector (Mock; Supplementary Fig. S4b ). To further investigate the role of JNK activity in CD146-promoted cell migration, CD146-HEK293T cells were pretreated with JNK inhibitor (10 μm SP600125) for 1 h. The motility of CD146-HEK293T cells was largely attenuated by the inhibition of JNK activity while mock-treated (dimethyl sulphoxide) cells migrated normally ( Fig. 2f ). These results suggest that CD146 promotes cell migration by activating JNK in the non-canonical Wnt signalling pathway. CD146 binds to Dvl2 and regulates the activation of Dvl2 Dvl2 is the scaffold protein that relays Wnt signalling by bridging receptor and adaptor proteins in both canonical and non-canonical Wnt pathways [25] , [26] . As CD146 was required for the activation of JNK by Wnt5a, we hypothesized that CD146 may relay Wnt signalling through Dvl. Co-IP indicated that CD146 physically interacts with Dvl2 ( Fig. 3a ). Interestingly, we found that the interaction between CD146 and Dvl2 was significantly enhanced in the presence of Wnt5a ( Fig. 3b ). Membrane translocation is critical for Dvl function in non-canonical Wnt signalling [27] . Immunostaining showed that the expression of Flag-tagged Dvl2 alone gave a punctate pattern and was evenly distributed in the cytoplasm. Partial co-localization of CD146 and Dvl2 on the cell membrane was detected in cells transfected with CD146 and Dvl2. Moreover, CD146 began to internalize and its co-internalization with Dvl2 was enhanced on Wnt5a treatment ( Supplementary Fig. S11 ). 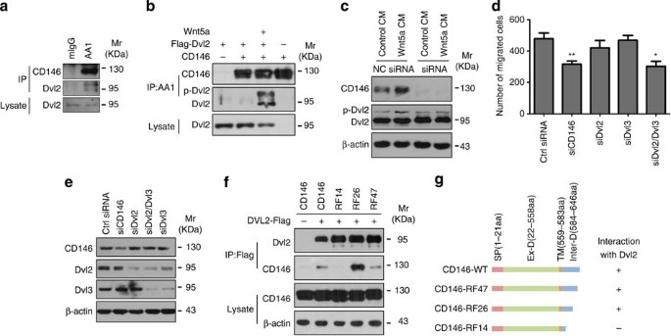Figure 3: CD146 interacts with Dvl and is required for Wnt-induced Dvl phosphorylation. (a) CD146 interacts with Dvl endogenously. HUVEC lysates were subjected to Co-IP with CD146 antibody AA1, mIgG being used as a negative control. The membrane was probed with anti-Dvl2 antibodies. (b) Wnt5a promotes the interaction between CD146 and Dvl2; Wnt5a CM was added to cells co-expressing CD146 and Dvl2 for 1 h. Cells were then collected and assayed by Co-IP. (c) Knockdown of CD146 blocks Wnt5a-induced Dvl2 phosphorylation; CD146-specific siRNA was used to knockdown endogenous CD146 in HUVECs. Wnt5a CM or control CM was added to induce Dvl2 phosphorylation. Bands of phosphorylated Dvl2 with larger molecular weights were detected by western blotting. β-actin was used as a loading control. (d) Knockdown of both Dvl2 and Dvl3 inhibits CD146-induced cell migration. The numbers of migrated cells were determined as described in the Methods. Data are presented as mean values±s.d. of three experiments. Significant difference was determined by Student’st-test (*P<0.05; **P<0.01). (e) Knockdown efficiency of Dvl2 and Dvl3 in CD146-HEK293T cells. (f) The 14–26 amino-acid region of the intracellular domain of CD146 is required for its interaction with Dvl2. A series of C-terminal truncations of CD146 at the intracellular domain were transfected with Dvl2. Co-IP was performed as described in the Methods. (g) Schematic diagram of the CD146 truncated forms and their interaction with Dvl2. Figure 3: CD146 interacts with Dvl and is required for Wnt-induced Dvl phosphorylation. ( a ) CD146 interacts with Dvl endogenously. HUVEC lysates were subjected to Co-IP with CD146 antibody AA1, mIgG being used as a negative control. The membrane was probed with anti-Dvl2 antibodies. ( b ) Wnt5a promotes the interaction between CD146 and Dvl2; Wnt5a CM was added to cells co-expressing CD146 and Dvl2 for 1 h. Cells were then collected and assayed by Co-IP. ( c ) Knockdown of CD146 blocks Wnt5a-induced Dvl2 phosphorylation; CD146-specific siRNA was used to knockdown endogenous CD146 in HUVECs. Wnt5a CM or control CM was added to induce Dvl2 phosphorylation. Bands of phosphorylated Dvl2 with larger molecular weights were detected by western blotting. β-actin was used as a loading control. ( d ) Knockdown of both Dvl2 and Dvl3 inhibits CD146-induced cell migration. The numbers of migrated cells were determined as described in the Methods. Data are presented as mean values±s.d. of three experiments. Significant difference was determined by Student’s t -test (* P <0.05; ** P <0.01). ( e ) Knockdown efficiency of Dvl2 and Dvl3 in CD146-HEK293T cells. ( f ) The 14–26 amino-acid region of the intracellular domain of CD146 is required for its interaction with Dvl2. A series of C-terminal truncations of CD146 at the intracellular domain were transfected with Dvl2. Co-IP was performed as described in the Methods. ( g ) Schematic diagram of the CD146 truncated forms and their interaction with Dvl2. Full size image Dvl phosphorylation is essential for Wnt signalling transduction. Phosphorylation of Dvl2 was increased markedly by Wnt5a ( Fig. 3b ). To further verify that CD146 is the receptor for Wnt5a in signalling transduction, we evaluated the phosphorylation of Dvl2 in HUVECs by knocking down CD146. Phosphorylated Dvl2 with larger molecular weight was enhanced on Wnt5a treatment ( Fig. 3c ). However, the phosphorylation of Dvl2 was blocked when CD146 was depleted using CD146-specific siRNA ( Fig. 3c ). To examine the role of Dvl2 in CD146-induced cell migration, different isoforms of Dvl were knocked down in CD146-HEK293T cells ( Fig. 3e ). Interestingly, knocking down Dvl2 or Dvl3 separately did not affect cell motility, but simultaneous depletion of both Dvl2 and Dvl3 significantly impaired cell motility compared with the control siRNA group ( Fig. 3d ), suggesting redundancy in the function of Dvl2 and Dvl3 in Wnt5a–CD146-regulated cell motility. Altogether, these results strongly suggest that CD146 is the receptor of Wnt5a and that it relays Wnt5a signalling through Dvl. The Dvl2-binding region is required for CD146-activating JNK To determine the region of CD146 that interacts with Dvl2, we generated a series of constructs truncated at the carboxy terminus of CD146 ( Fig. 3g ). Co-IP results showed that the cytoplasmic region (14–26 amino acids) of CD146 is critical for its interaction with Dvl2 ( Fig. 3f,g ). Mutant CD146-RF14 (CD146 with 14 amino acids of the intracellular region remaining) lost its capacity to interact with Dvl2, whereas RF26 (with 26 amino acids of the intracellular region remaining) was still able to bind Dvl2. Binding between RF26 and Dvl2 was even stronger than that between wild-type (WT) CD146 and Dvl2, suggesting that the 14–26 amino acid intracellular region of CD146 is critical for its interaction with Dvl2. As CD146 regulates cell motility by activating non-canonical Wnt/Dvl/JNK signalling ( Fig. 2d,e ), we evaluated the signalling induction and biological functions of the above mutants ( Fig. 3g ). JNK was highly activated by WT CD146 and the positive control Dvl2. RF26 was able to interact with Dvl2, retaining its capacity to activate JNK. Other truncated forms, such as RF14 or the ECD of CD146 with a mutated Dvl2-binding region, failed to activate JNK ( Fig. 4a ). 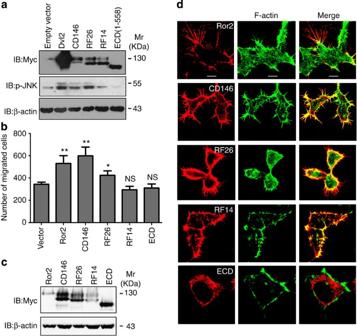Figure 4: The effect of CD146 and its truncated forms on cell migration and the formation of cell protrusions. (a) Different CD146 mutants activate JNK. Two micrograms of each plasmid (Fig. 3g) was transfected into HEK293T cells for 36 h, and JNK activity was measured with p-JNK antibodies. β-actin was used as a loading control. (b,c) Different mutants of CD146 promote cell migration. The CD146 mutants depicted inFig. 3gwere transiently transfected into HEK293T cells for 36 h. Five thousand transfected cells were seeded in transwell plates, and migrated cells were counted. The expression of CD146 mutants was determined by western blotting. Data shown are representative of experiments repeated three times. Ror2 was used as a positive control. Data are presented as mean values±s.d. of three experiments. Significant difference was determined by Student’st-test (*P<0.05; **P<0.01; NS, no significant difference). (d) CD146 mutants induce cell polarity. Different CD146 mutants were transfected into HEK293T cells for 36 h and cells were then stained with AA1 and F-actin. Images were taken with a confocal microscope. Ror2 was used as a positive control (scale bar, 10 μm). Figure 4: The effect of CD146 and its truncated forms on cell migration and the formation of cell protrusions. ( a ) Different CD146 mutants activate JNK. Two micrograms of each plasmid ( Fig. 3g ) was transfected into HEK293T cells for 36 h, and JNK activity was measured with p-JNK antibodies. β-actin was used as a loading control. ( b , c ) Different mutants of CD146 promote cell migration. The CD146 mutants depicted in Fig. 3g were transiently transfected into HEK293T cells for 36 h. Five thousand transfected cells were seeded in transwell plates, and migrated cells were counted. The expression of CD146 mutants was determined by western blotting. Data shown are representative of experiments repeated three times. Ror2 was used as a positive control. Data are presented as mean values±s.d. of three experiments. Significant difference was determined by Student’s t -test (* P <0.05; ** P <0.01; NS, no significant difference). ( d ) CD146 mutants induce cell polarity. Different CD146 mutants were transfected into HEK293T cells for 36 h and cells were then stained with AA1 and F-actin. Images were taken with a confocal microscope. Ror2 was used as a positive control (scale bar, 10 μm). Full size image CD146–Dvl2 interaction regulates cell motility We next evaluated the ability of these mutants to induce cell migration by transiently transfecting each mutant into HEK293T cells. We found that WT CD146 promoted significantly more cells to migrate, comparable to Ror2. Both RF14 and the ECD of CD146, which have lost their Dvl2-binding ability, failed to mediate cell migration, indicating that binding Dvl2 is critical for CD146-induced cell migration ( Fig. 4b,c ). Together, these results indicate that the activation of non-canonical Wnt JNK signalling and promotion of cell migration by CD146 are dependent on the interaction between Dvl2 and CD146. CD146 promotes the formation of cell protrusions To explore whether the subcellular localization of CD146 or Wnt4 receptors, such as Ror2, Fz5 or Fz7, was altered in the presence/absence of Wnt5a, immunostaining assays were performed. Results suggest that in the presence of Wnt5a, the subcellular localization of CD146 is altered. CD146 was accumulated on the cell membrane, in a specific region, thus displaying a polarized enrichment of actin filaments as reported [28] . However, alteration in localization of Ror2, Fz5 or Fz7 was not observed in the presence of Wnt5a ( Supplementary Fig. S12 ). Non-canonical Wnt signalling mainly regulates tissue cell migration and cell polarity. Cell polarity characterized by the protrusion of F-actin is the main driving force for cell migration [8] . Myc-tagged CD146 (Myc-CD146) was used to transfect HEK293T, MCF-7 and SW480 cell lines. Surprisingly, ectopic expression of CD146 alone without Wnt5a stimulation promoted filopodia formation, as demonstrated by 488-phalloidin staining ( Fig. 4d ). Imaging data showed that CD146, like Ror2, is localized at the protrusion and promotes the formation of cell protrusions. Mutant RF14 is still localized with F-actin, but barely promoted the formation of cell protrusions ( Fig. 4d ), whereas the ECD of CD146 was not localized with F-actin and failed to promote the formation of cell protrusions. RF26 seems to be less able to promote cell migration and formation of cell protrusion than WT CD146 ( Fig. 4b,d ). It might be due to either the lack of the deleted region or a conformational change that is involved in the function of CD 146 on cell migration and protrusion. These results suggest that CD146 promotion of the formation of cell protrusions is largely dependent on its binding of Dvl [29] , consistent with previous results showing that CD146-mediated cell migration and JNK activity are also Dvl binding-dependent. CD146 regulates CE movement during zebrafish gastrulation To further investigate the role of CD146 in regulating cell migration, we used zebrafish embryos to explore the role of CD146 during embryo gastrulation when cells undergo extensive CE movement. CD146 is maternally expressed from the one-cell stage and ubiquitously expressed until bud stage as demonstrated by whole-mount in situ hybridization (WISH; Supplementary Fig. S13 ). CD146 was expressed in somites and lateral mesoderm at the 10- and 18-somite stages and in vascular endothelial cells at 24 hours post fertilization (hpf; Supplementary Fig. S13 ). We designed a translation-blocking morpholino oligonucleotide (MO) against CD146, and found that expression of CD146, as detected by western blotting, was efficiently suppressed ( Fig. 5c ). Approximately 95% of embryos ( n >50) injected with 50 pg CD146 messenger RNA or 4 ng MO, like Wnt5a-injected embryos, exhibited an increased angle between their anterior and posterior ends, and widened notochord or irregular somites ( Fig. 5a,b ). These phenotypes are commonly associated with gastrulation defects caused by impaired CE and PCP signalling. We next examined the expression pattern of CE movement marker genes, including hgg , dlx3 , ntl and myoD ( Fig. 5b ). Compared with control embryos, the expression patterns of these genes were altered in embryos injected with either CD146 MO or mRNA. Interestingly, gsc , a neuroectoderm marker, showed a normal expression pattern, indicating that cell fate had not been changed. 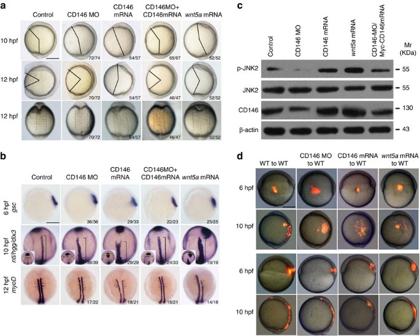Figure 5: CD146 is required for CE during zebrafish gastrulation. (a) CD146 is essential for CE movement. Embryos at the one-cell stage were injected with 0.5 nM control MO, 4 ng CD146 MO, 50 pg N-terminal Myc-CD146 mRNA and 50 pg Wnt5a mRNA or with CD146 MO plus Myc-CD146 mRNA. These embryos were either viewed laterally, anterior to the top, at 10 hpf and 12 hpf or viewed from the dorsal side at 12 hpf. The angle between the anterior end and the posterior end was measured (scale bar, 250 μm). (b) Knockdown or overexpression of CD146 affects the expression of CE movement-related genes as determined by WISH. The expression pattern of the neuroectoderm markergscwas determined by WISH at 6 hpf and that of the pre-chordal plate markerhgg1, neuroectoderm markerdlx3and notochord markerntlwere determined at 10 hpf. The expression pattern of the somite markermyoDwas determined at 12 hpf (scale bar, 250 μm). (c) Knockdown of CD146 inhibits JNK activity. Embryos were collected at 10 hpf after injection with control MO, CD146 MO, Myc-CD146 mRNA, Wnt5a mRNA or Myc-CD146 mRNA plus CD146 MO. The expression level of CD146, JNK2 and p-JNK2 was determined by western blotting. β-actin was used as a loading control. (d) CD146 regulates CE movement cell autonomously. Lateral (top two panels) or axial (bottom two panels) cells (red) derived from control, CD146 MO, CD146 mRNA or Wnt5a-mRNA-injected embryos at the shield stage (6 hpf) were transplanted into the corresponding regions of WT recipients at the shield stage and then collected and analysed at the bud stage (10 hpf; scale bar, 250 μm). Figure 5: CD146 is required for CE during zebrafish gastrulation. ( a ) CD146 is essential for CE movement. Embryos at the one-cell stage were injected with 0.5 nM control MO, 4 ng CD146 MO, 50 pg N-terminal Myc-CD146 mRNA and 50 pg Wnt5a mRNA or with CD146 MO plus Myc-CD146 mRNA. These embryos were either viewed laterally, anterior to the top, at 10 hpf and 12 hpf or viewed from the dorsal side at 12 hpf. The angle between the anterior end and the posterior end was measured (scale bar, 250 μm). ( b ) Knockdown or overexpression of CD146 affects the expression of CE movement-related genes as determined by WISH. The expression pattern of the neuroectoderm marker gsc was determined by WISH at 6 hpf and that of the pre-chordal plate marker hgg1 , neuroectoderm marker dlx3 and notochord marker ntl were determined at 10 hpf. The expression pattern of the somite marker myoD was determined at 12 hpf (scale bar, 250 μm). ( c ) Knockdown of CD146 inhibits JNK activity. Embryos were collected at 10 hpf after injection with control MO, CD146 MO, Myc-CD146 mRNA, Wnt5a mRNA or Myc-CD146 mRNA plus CD146 MO. The expression level of CD146, JNK2 and p-JNK2 was determined by western blotting. β-actin was used as a loading control. ( d ) CD146 regulates CE movement cell autonomously. Lateral (top two panels) or axial (bottom two panels) cells (red) derived from control, CD146 MO, CD146 mRNA or Wnt5a-mRNA-injected embryos at the shield stage (6 hpf) were transplanted into the corresponding regions of WT recipients at the shield stage and then collected and analysed at the bud stage (10 hpf; scale bar, 250 μm). Full size image To confirm that the phenotype caused by CD146-MO was specific, we co-injected CD146 MO with N-terminal Myc-CD146 mRNA into zebrafish embryos at the one-cell stage. Both phenotype and expression of CE movement markers in MO-injected embryos were rescued by co-injection with Myc-CD146 mRNA ( Fig. 5a,b ). In addition, the phosphorylation of JNK2, a marker of the Wnt/PCP pathway during CE movement, was suppressed in embryos in which CD146 was knocked down ( Fig. 5c ). These data are consistent with our observations in mammalian cells. To further clarify whether CD146 regulates CE movement cell autonomously, we performed cell transplantation experiments. Lateral mesendodermal cells from the lateral blastoderm margin of WT, CD146 MO, Myc-CD146 and Wnt5a-mRNA-injected embryos were transplanted into the corresponding regions of WT recipients at the shield stage. After gastrulation, cells donated from WT embryos migrated to the dorsal side, while this convergence movement was delayed in CD146-deficient, CD146 and Wnt5a-overexpressing donor cells ( Fig. 5d ). We then examined extension movements by transplanting axial mesendodermal cells from the donor embryos into the shield of WT recipients. Compared with controls, CD146-deficient, CD146 and Wnt5a-overexpressing donor cells showed blocked or delayed extension movements in WT recipients. Taken together, these results demonstrate that CD146 regulates CE movements in a cell-autonomous manner. CD146 inhibits canonical Wnt signalling at β-catenin level To analyse the role of CD146 in regulating canonical Wnt signalling, we employed a TCF transcription activity assay [30] . Our results indicated that CD146 inhibits canonical Wnt signalling in a dose-dependent manner in HEK293T cells ( Fig. 6a , Supplementary Fig. S14a ). Conversely, knockdown of CD146 in CD146-HEK293T significantly enhanced canonical Wnt signalling ( Fig. 6b ). To investigate at which step CD146 exerts its inhibitory effect in this pathway, various doses of CD146 were co-transfected with different components of the canonical Wnt pathway. Results showed that CD146 not only inhibits receptor (Fz8) and co-receptor (Lrp6)-activated canonical Wnt signalling ( Supplementary Fig. S14c,d ), but also inhibits scaffold protein Dvl2-activated canonical Wnt signalling in a dose-dependent manner ( Supplementary Fig. S14e ). The mutant β-catenin/S37A (Ser 37 was substituted by Ala) is a relatively stable form of β-catenin [31] . CD146 inhibited WT β-catenin but not β-catenin/S37A-activated Wnt signalling in a dose-dependent manner ( Fig. 6c ). These results, therefore, strongly suggest that CD146 inhibits canonical Wnt signalling at the β-catenin level. 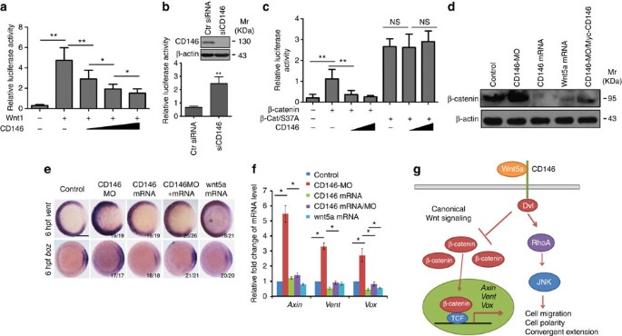Figure 6: CD146 inhibits canonical Wnt signalling at the β-catenin level. (a) CD146 inhibits Wnt1 signalling in a dose-dependent manner, as determined by luciferase reporter assays in HEK293T cells. Data are presented as mean values±s.d. of three experiments. Significant difference was determined by Student’st-test (*P<0.05; **P<0.01). (b) Knockdown of CD146 promotes canonical Wnt-activated TCF transcription as determined by luciferase reporter assays in CD146-HEK293T. Data are presented as mean values±s.d. of three experiments. Significant difference was determined by Student’st-test (**P<0.01). (c) CD146 inhibits only WT β-catenin but not mutant β-catenin/S37A-activated signalling in a dose-dependent manner. Data are presented as mean values±s.d. of three experiments. Significant difference was determined by Student’st-test (**P<0.01; NS, no significant difference). (d) The protein level of β-catenin is negatively correlated with CD146 expression in zebrafish embryos. Embryos were injected with CD146 mRNA and/or MO as indicated and collected at 6 hpf. Proteins were subjected to western blotting, Wnt5a was used as a positive control. β-actin was used as a loading control. (e) CD146 is negatively correlated with β-catenin target genes in zebrafish embryos as shown byin situhybridization. The expression patterns of the dorsal-ventral patterning markersventandbozwere determined in embryos injected with CD146 morphant, CD146 mRNA or Wnt5a mRNA, or a combination of CD146 MO and Myc-CD146 mRNA at 6 hpf (scale bar, 250 μm). (f) CD146 is negatively correlated with β-catenin target gene expression in zebrafish embryos as shown by real-time PCR. The injected embryos were collected at 6 hpf, and β-catenin target genesAxin,VentandVoxwere analysed by real-time PCR. All bars represent the mean values±s.d. of three experiments. Significant difference was determined by Student’st-test (*P<0.05). (g) A model of the regulatory pattern of CD146 in canonical and non-canonical Wnt signalling. See text for details. Figure 6: CD146 inhibits canonical Wnt signalling at the β-catenin level. ( a ) CD146 inhibits Wnt1 signalling in a dose-dependent manner, as determined by luciferase reporter assays in HEK293T cells. Data are presented as mean values±s.d. of three experiments. Significant difference was determined by Student’s t -test (* P <0.05; ** P <0.01). ( b ) Knockdown of CD146 promotes canonical Wnt-activated TCF transcription as determined by luciferase reporter assays in CD146-HEK293T. Data are presented as mean values±s.d. of three experiments. Significant difference was determined by Student’s t -test (** P <0.01). ( c ) CD146 inhibits only WT β-catenin but not mutant β-catenin/S37A-activated signalling in a dose-dependent manner. Data are presented as mean values±s.d. of three experiments. Significant difference was determined by Student’s t -test (** P <0.01; NS, no significant difference). ( d ) The protein level of β-catenin is negatively correlated with CD146 expression in zebrafish embryos. Embryos were injected with CD146 mRNA and/or MO as indicated and collected at 6 hpf. Proteins were subjected to western blotting, Wnt5a was used as a positive control. β-actin was used as a loading control. ( e ) CD146 is negatively correlated with β-catenin target genes in zebrafish embryos as shown by in situ hybridization. The expression patterns of the dorsal-ventral patterning markers vent and boz were determined in embryos injected with CD146 morphant, CD146 mRNA or Wnt5a mRNA, or a combination of CD146 MO and Myc-CD146 mRNA at 6 hpf (scale bar, 250 μm). ( f ) CD146 is negatively correlated with β-catenin target gene expression in zebrafish embryos as shown by real-time PCR. The injected embryos were collected at 6 hpf, and β-catenin target genes Axin , Vent and Vox were analysed by real-time PCR. All bars represent the mean values±s.d. of three experiments. Significant difference was determined by Student’s t -test (* P <0.05). ( g ) A model of the regulatory pattern of CD146 in canonical and non-canonical Wnt signalling. See text for details. Full size image After receiving canonical Wnt signalling, β-catenin is stabilized in the cytosol, and then translocates into the nucleus where it binds to the promoter of TCF/Lef to regulate the expression of target genes. Further analysis indicated that CD146 promotes native or Wnt1-activated β-catenin degradation in the cytosol, ( Supplementary Fig. S14b,f ). This was verified by injecting CD146 mRNA into zebrafish embryos. Conversely, knockdown of CD146 stabilizes β-catenin in embryos ( Fig. 6d ). As a consequence, the expression of the target genes of β-catenin, vent or boz , was upregulated in CD146 morphants. Conversely, the expression of these genes was downregulated in embryos injected with CD146 mRNA, as determined by in situ hybridization ( Fig. 6e ). This negative correlation between CD146 and β-catenin was also observed by examining the mRNA levels of Axin , Vent and Vox , the target genes of β-catenin, in embryos by real-time PCR ( Fig. 6f ). These results strongly suggest that CD146 is a negative regulator of canonical Wnt signalling at the β-catenin level. Non-canonical Wnt signalling has a pivotal role in regulating cell motility, cell polarity and CE during embryo gastrulation. Here we identified CD146 as a receptor of Wnt5a in the regulation of non-canonical Wnt signalling. Knockdown of CD146 inhibits Wnt5a-induced cell migration and JNK activity. Depletion of CD146 with MO impairs CE in zebrafish, leading to gastrulation defects in embryos. Further, CD146 relays Wnt5a signalling through Dvls, as knockdown of CD146 blocks Wnt5a-induced Dvl2 phosphorylation. Indeed, CD146 physically interacts with Dvl2. Knockdown of Dvl2 and Dvl3 attenuates CD146-induced cell migration. The 14–26 amino-acid region of the intracellular domain of CD146 is important for their interaction. Interestingly, CD146 also regulates canonical Wnt signalling by inhibiting its signalling at the β-catenin level. Although CD146 has been extensively studied in tumour metastasis, invasion and angiogenesis, its ligand is still under investigation [16] , [32] , [33] , [34] . As a non-canonical Wnt ligand, Wnt5a has a critical role in regulating cell motility, cell polarity and CE during embryo gastrulation. Polarized redistribution of CD146 has been reported in the regulation of cell migration and cell polarity via recruitment of actin and myosin on Wnt5a treatment. Here we provide evidence that CD146 is a non-canonical Wnt5a receptor in the regulation of cell motility, cell polarity and CE during zebrafish gastrulation. CD146 binds Wnt5a with high affinity, comparable to that of the known Wnt receptor Fz5 ( Fig. 1a–c ). The subcellular localization of CD146 was altered in the presence of Wnt5a, which accumulates in the cell membrane, at a specific region that displays a polarized enrichment of actin filaments ( Supplementary Fig. S12 ) [28] . However, a change in localization in the presence of Wnt5a has not been observed for Ror2, Fz5 or Fz7 ( Supplementary Fig. S12 ). Similarly, localization or expression levels of these Wnt receptors were not altered when expression of CD146 was modulated ( Supplementary Figs S9 and S10 ). These results indicate that CD146 regulates Wnt signalling without affecting the expression of other Wnt receptors such as Ror2, Fz5 and Fz7. Similar to most of the genes identified in the Wnt/PCP pathway, knockdown of CD146 impairs cell motility and CE movement during gastrulation [35] ( Figs 2a and 5a ). The phenotype of CD146 morphant embryos is similar to that of Wnt5a morphants with wider and shorter notochord accompanying a wider and disordered somites ( Fig. 5a,b ) [36] . These phenotypes commonly result from impaired Wnt/PCP signalling in association with gastrulation defects [35] . Further analysis indicates that the third Ig-like region of CD146 (236–321 amino acids) is required for Wnt5a binding ( Fig. 1d,e ). The (322–646 amino acids/CD146) mutant can efficiently rescue the phenotype and reduce the increased canonical Wnt signalling in CD146 MO morphants ( Supplementary Fig. S15 ). However, we did not observe the rescue effect in non-canonical Wnt signalling ( Supplementary Fig. S16 ). Cell adhesion assay indicates that the (322–646 amino acids/CD146) mutant still exhibits strong cell adhesion activity compared with that of full-length CD146, suggesting that Wnt5a signalling is important for CD146 morphogenetic activity ( Supplementary Figs S6b and S16 ). To clarify whether CD146 also binds other Wnt ligands, Wnt1 or Wnt3a were co-expressed with CD146 in HEK293T cell. Results showed that CD146 binds to canonical Wnt ligands such as Wnt1 and Wnt3a ( Supplementary Fig. S2a,b ). Similar to Ror2, which binds to canonical Wnt ligands, CD146 mainly activates non-canonical Wnt signalling. The specificity of Wnt signalling might depend on the endogenous expression of individual ligands or receptors in a cell context-dependent manner [10] . However, how, when and where Wnt ligands use different receptors to distinguish the canonical and non-canonical branches warrants further investigation. Among the different branches of the non-canonical Wnt pathway, such as the Wnt/Dvl/JNK (PCP) pathway, Wnt/Ca2 + and Wnt/Ror2 pathways, the PCP pathway is the best defined [37] . CD146 activates JNK extensively in different cell types ( Fig. 2e ). As a receptor of Wnt5a, CD146 is required for Wnt5a-activated JNK signalling and cell migration. Knockdown of CD146 decreases the baseline level of p-JNK both in vitro and in vivo ( Figs 2b and 5c ). On the other hand, CD146 alone may not fully activate JNK, as knockdown of Fz4 impairs JNK activity ( Supplementary Fig. S7 ), suggesting that CD146 may cooperate with other Wnt receptors in regulating non-canonical Wnt signalling. Further, antibodies against the ECD of CD146 can block Wnt5a-induced cell migration and JNK activity ( Fig. 2c,d ), probably by interfering with the interaction between CD146 and Wnt5a( Supplementary Fig. S5 ).Wnt5a may slightly inhibit cell adhesion possibly through downregulation of the adhesion molecule β-catenin and its target genes, such as E-cadherin ( Supplementary Fig. S6a ) [38] . Moreover, JNK inhibitor SP600125 attenuates CD146-promoted cell motility ( Fig. 2e ). We have previously reported that CD146 promotes melanoma cell migration by activating small GTPase RhoA [18] . RhoA is an important component of the non-canonical Wnt pathway located downstream of Dvls. Accordingly, RhoA is critical for activating JNK in the regulation of cell motility and the formation of cell protrusions [37] . As a scaffold protein in the Wnt pathway, Dvl functions in both canonical and non-canonical Wnt pathways. Phosphorylation and membrane translocation are critical for Dvl function in the non-canonical Wnt pathway. In the presence of the Wnt ligand, Dvl is phosphorylated and recruited by its receptor to the cell membrane, switching Wnt signalling from the canonical to the PCP pathway [39] . Interactions between CD146 and Dvl2 and the phosphorylated form of Dvl2 increase in the presence of Wnt5a ( Fig. 3b ). Indeed, enhanced co-localization of CD146 and Dvl2 at the cell membrane was observed under Wnt5a treatment ( Supplementary Fig. S11 ). Further analysis showed that the 14–26 amino-acid region of the intracellular domain is critical for CD146 binding with Dvl2 ( Fig. 3f ). This region is also critical for CD146 activation of JNK, promoting cell migration and the formation of protrusions ( Fig. 4a–d ). In addition, knockdown of Dvls attenuates CD146-promoted cell migration ( Fig. 3d,e ). Here we have demonstrated that CD146 regulates non-canonical Wnt signalling by activating JNK via Dvl to promote cell motility and cell polarity. We previously reported that CD146 regulates melanoma cell migration by regulating the binding protein actin-linking ezrin-radixin-moesin (ERM) [18] . Although ERM and Dvl both bind to CD146 at its cytoplasmic tail, their interaction with CD146 displays different properties: first, ERM binds to the positively charged region (KKGK) of CD146, whereas Dvl binds to a different region close to the KKGK motif; second, the binding of CD146 to ERM is constitutive. However, the binding of CD146 to Dvl is very weak in absence of Wnt5a but is enhanced in the presence of Wnt5a. As a ligand of the non-canonical Wnt pathway, Wnt5a inhibits canonical Wnt signalling in a receptor-dependent manner [40] . Similarly, an inhibitory role of CD146 in canonical Wnt signalling has been observed ( Fig. 6 ). Accordingly, depletion of CD146 enhanced Wnt1-activated TCF transcription ( Fig. 6b ). The inhibitory effect of CD146 was observed at the β-catenin level ( Fig. 6c ). Indeed, β-catenin protein was markedly downregulated or upregulated by overexpression or knockdown of CD146, respectively, both in vitro and in vivo ( Fig. 6 ). As a result, the target genes of β-catenin were upregulated or downregulated by the knockdown or overexpression of CD146 in zebrafish embryos, respectively ( Fig. 6e,f ). Moreover, this negative correlation between CD146 and β-catenin at the protein level was also observed in different colon cancer cell lines ( Supplementary Fig. S17 ), implying the involvement of CD146 in colon cancer. We have previously reported that CD146 induces the epithelial–mesenchymal transition by downregulating the expression of E-cadherin in breast cancer cell lines [16] . E-cadherin, an adhesion molecule anchoring β-catenin to the cell membrane, has been identified as a canonical Wnt target gene and is positively regulated by Wnt [41] , [42] . In this study, we demonstrate that CD146 is the negative regulator of canonical Wnt signalling. CD146 may decrease the level of E-cadherin by downregulating β-catenin. The balance between canonical and non-canonical Wnt signalling is tightly controlled. Identification of the Wnt5a/CD146 pathway in this study provides new insights for explaining why the non-canonical ligand Wnt5a can inhibit canonical Wnt signalling. However, the exact mechanism by which CD146 destabilizes β-catenin and inhibits canonical Wnt signalling still needs further investigation. Recently, several atypical adhesion molecules (Fat, Dachsous and Flamingo) have been identified as non-canonical Wnt receptors in the Wnt/Dvl/JNK pathway, which is involved in regulating cell motility and cell polarity, indicating that adhesion molecules have an important role in mediating the Wnt signalling pathway [43] . However, whether these adhesion molecules and CD146 have synergistic roles in regulating Wnt signalling remain to be explored. In summary, we have identified CD146 as a Wnt5a receptor that simultaneously activates non-canonical Wnt signalling and inhibits canonical Wnt signalling as depicted in Fig. 6g . Our results may help provide clearer understanding of the roles of adhesion molecules in regulating the cell motility and cell polarity that are essential in both normal development and tumour pathogenesis. Our findings may also provide new markers for cancer diagnosis and new targets for cancer treatment, especially for metastatic tumours. Antibodies and reagents Anti-CD146 rabbit polyclonal antibody, monoclonal antibodies AA1, AA2, AA3 and AA98 were generated in our laboratory [44] . Anti-FLAG (F1804, 1:3,000) and anti-β-actin (AC15, 1:5,000) antibodies were from Sigma-Aldrich (St Louis, MO, USA). Anti-Dvl3 antibody(sc-8027, 1:1,000) was from Santa Cruz Biotechnology (Santa Cruz, CA, USA). Anti-Dvl2 (#3216, 1:1,000), Anti-Myc (#2276, 1:5,000 for western, 1:500 for immunostaining), JNK (#9252, 1:1,000), anti-β-catenin (#610514, 1:5,000) and p-JNK/SPARK (#4668, 1:1,000) antibodies were purchased from Cell Signaling (Danvers, MA, USA). Anti-Ror2 (ab92379, 1:1,000), Fz7 (ab64636, 1:1,000) and Fz5 (ab14475, 1:1,000) antibodies were obtained from Abcam. Fast red tablets were obtained from Roche (Basel, Switzerland). Cell adhesion assay kit (extracellular matrix array) was obtained from Cell BioLabs. Fc and Fc-CD146 were from Sino Biological, and recombinant human Wnt5a were obtained from R&D Systems. Plasmids and siRNA Flag-CD146 , Myc-CD146 and Myc-Wnt5a were generated by PCR and cloned into N-terminal Flag or Myc-tagged PCS2-sp empty vectors digesting with Hind III at N terminal and Bgl II at C terminal; Flag-hFz8 , Flag-hFz5 , Flag- xFz7 , Myc- hFz5 , Myc- xFz7 , Flag-hGSk3ß , Flag-β-Catenin , Flag-β-Catenin-S37A and luciferase reporter plasmids were kindly provided by Dr Wei Wu (Tsinghua University). Different constructs for N-terminal-truncated CD146 were generated by PCR and cloned into PCS2-sp-Flag with Eco RI at N terminal and Bgl II at C terminal and verified by sequence. Small interfering RNA (siRNA) targeting CD146, Dvl2, Dvl3, Ror2, Fz2, Fz3, Fz4, Fz5, Fz6, Fz7 and control siRNA were synthesized by Invitrogen (San Diego, CA, USA) using previously reported sequences as listed in Supplementary Table S1 (refs 23 , 32 , 45 , 46 ). Transfection and luciferase reporter assays HEK293T, SW480, HUVEC and HT-29 cells were plated in 10 cm dishes or six-well plates. Cells were transfected with 50 nM siRNAs or plasmids using Fugene-6 transfection reagent (Roche). HEK293T and HUVECs used in the luciferase reporter assay were seeded in 48-well plates and transfected in triplicate with plasmids or siRNAs together with Super TOP-FLASH . pRL-TK was used as an internal control and luciferase activity was determined as described [30] . The amount of plasmid used per well was as follows: 15 ng of Super TOP-FLASH , 0.5 ng of pRL-TK , 10 ng of Lrp6 , 10 ng of Frizzled , 10 ng of Wnt1 , 10 ng of Dvl , 10 ng of β-catenin or the mutant β-catenin/S37A. Cell surface-binding assay Myc-Wnt5a was transfected into HEK293T cells for 48 h, and then the cell culture medium (Wnt5a CM) was collected and concentrated with Amicon-Ultra-15 filters (Millipore). CD146 , Fz5 , Fz7 or an empty vector were transfected into HEK293T cells for 36 h and the cell surface-binding assay was performed as described [19] . Enzyme-linked immunosorbent assay-based binding curve Fc (0.4 mg ml −1 ), Fc-CD146 or Fc-Fz5 was coated on 96-well plates overnight at 4 °C; 0.625–40 nM of Wnt5a or Wnt3a (determined by western blotting) were then added into the Fc-, CD146- or Fz5-coated wells and incubated for 3 h at room temperature. Mouse anti-Myc primary antibody, horseradish peroxidase-conjugated goat-anti-mouse secondary antibody and horseradish peroxidase substrate were then sequentially added to the wells and incubated 1 h. Absorbance values were then read at OD450 (ref. 47 ). Co-IP assays and immunoblotting For immunoprecipitation, cells in six-well plates were lysed on ice with TNE buffer (10 mM Tris, pH 7.4, 150 mM NaCl, 0.5% NP-40, 1 mM EDTA) supplemented with 2 mM sodium vanadate, 25 mM sodium fluoride and a protease inhibitor cocktail 40 h post-transfection. FLAG- or Myc-tagged proteins were recovered using anti-FLAG agarose beads (M2; Sigma) or protein A/G plus CD146 antibody AA1, respectively. For the pull-down assay, Fc-CD146/ECD, Fc-Fz5/ECD or Fc (100 ng ml −1 each) was conjugated with protein A beads and incubated with recombinant Wnt5a for 1 h. Bound proteins were eluted with loading buffer and analysed by immunoblotting. Full scans of western blots are supplied in Supplementary Fig. S18 . For cell fractionation, the cell membrane and cytosol were separated as described [48] . The resultant supernatant was taken as the cytosol fraction and analysed by immunoblotting. Immunoblotting was performed as described previously with antibodies against FLAG, Myc, β-catenin, Dvl2, Dvl3 JNK, p-JNK and mouse anti-CD146 antibody AA1 or rabbit anti-CD146 antibody [32] . Immunostaining For immunofluorescence, cells seeded on coverslips in six-well plates were fixed with 4% paraformaldehyde and permeabilized with 0.2% Triton X-100 in PBS buffer, and then blocked with PBS containing 3% BSA before addition of a primary antibody and secondary antibody (goat anti-rabbit-Alexa Fluor 488 or donkey anti-mouse-Alexa Fluor 568). Cell migration and adhesion assays Cell migration capacity was evaluated using the Transwell system [32] . In brief, 5,000 serum-starved cells in 100 μl of serum-free RPMI-1640 were added into the upper chamber and cultured with Wnt5a CM or control CM. Cells were allowed to migrate for 10 h and migrated cells were then counted. Cell adhesion ability was evaluated with the Cytoselect Cell adhesion assay Kit from Cell BioLabs. In brief, 10 6 of cells in serum-free RPMI-1640 were added onto the extracellular matrix protein-coated wells with 200 ng ml −1 Wnt5a or vehicle. After growing for 1 h, the adherent cells were captured and unbound cells were removed with consecutive washes. The adhesion cells were lysed and subsequently detected with CyQuant GR Dye. Experiments were carried out in triplicate. Fish strains Zebrafish embryos were obtained from adult Tubingen strain fish by natural spawning. Embryos were raised and maintained at 28.5 °C in system water and staged morphologically [49] . Morpholinos and mRNA synthesis CD146 MO (5′-AGCAGTGCGGTGTAGGTCATTTCTC-3′) and CD146 mismatch MO (5′-AGGCGTGCGGAGTAGCTCATTTGTC-3′) were obtained from GeneTools (Philomath, OR) and prepared as 1 mM stock solutions using double-distilled H 2 O. For CD146 knockdown experiments, 4 ng of CD146 MO was injected per embryo and embryos injected with CD146 mismatch MO at the same dosage were used as controls. hCD146 or xWnt5a mRNAs for injection were synthesized in vitro using an mMessage mMachine SP6 kit (Ambion) according to the manufacturer’s instructions. 50 pg of Myc-hCD146 mRNA, 50 pg of Wnt5a mRNA or 5 ng of CD146 MO per embryo was injected into zebrafish embryos at the one-cell stage. Whole-mount in situ hybridization WISH of zebrafish embryos was performed as described previously using the following probes: gsc , hgg , dlx3 , ntl , myoD , vent and boz [49] . Quantitative reverse transcriptase–PCR Total RNA was extracted from mammalian cells (HEK293T or HUVECs) or embryos (100 embryos were pooled for each sample) at the shield stage (6 hpf) using TriReagent (Tiangen, Beijing) and then reversely transcribed. The complementary DNAs were diluted five times to be used as templates. PCR was performed to amplify Wnt receptors with primers listed in Supplementary Table S2 or quantitative PCR was performed using the GoTaq qPCR Master Mix (Promega) on the Bio-Rad CFX96 Real-Time PCR system with primers against zebrafish Vent , Axin2 or Vox [49] listed in Supplementary Table S3 . Cell transplantation Donor embryos in the cell-autonomous assay were first co-injected at the one-cell stage with 1 nl of rhodamine-dextran (molecular weight 70,000WM; Molecular Probes) together with 4 ng of CD146 MO or 50 pg of CD146 or Wnt5a mRNA. Lateral or axial mesendodermal cells (30–50 cells) from the donor embryos were transplanted into the lateral margin or embryonic shield of WT hosts of the same developmental stage (shield stage, about 6 hpf). Images were obtained at 10 hpf under a microscope. Statistical analysis Statistical significance was calculated using Prism (GraphPad Software). All experiments were performed in triplicate. Data are shown as mean values±s.d. Statistical differences were determined with unpaired Student t- tests and P -values <0.05 were considered to be statistically significant. How to cite this article: Ye Z. D. et al. Wnt5a uses CD146 as a receptor to regulate cell motility and convergent extension. Nat. Commun. 4:2803 doi: 10.1038/ncomms3803 (2013).